Genesis of electron deficient Pt1(0) in PDMS-PEG aggregates While numerous single atoms stabilized by support surfaces have been reported, the synthesis of in-situ reduced discrete metal atoms weakly coordinated and stabilized in liquid media is a more challenging goal. We report the genesis of mononuclear electron deficient Pt 1 (0) by reducing H 2 PtCl 6 in liquid polydimethylsiloxane-polyethylene glycol (PDMS-PEG) (Pt 1 @PDMS-PEG). UV–Vis, far-IR, and X-ray photoelectron spectroscopies evidence the reduction of H 2 PtCl 6 . CO infrared, and 195 Pt and 13 C NMR spectroscopies provide strong evidence of Pt 1 (0), existing as a pseudo-octahedral structure of (R 1 OR 2 ) 2 Pt(0)Cl 2 H 2 (R 1 and R 2 are H, C, or Si groups accordingly). The weakly coordinated (R 1 OR 2 ) 2 Pt(0)Cl 2 H 2 structure and electron deficient Pt 1 (0) have been validated by comparing experimental and DFT calculated 195 Pt NMR spectra. The H + in protic state and the Cl − together resemble HCl as the weak coordination. Neutralization by a base causes the formation of Pt nanoparticles. The Pt 1 @PDMS-PEG shows ultrahigh activity in olefin hydrosilylation with excellent terminal adducts selectivity. Supported single atoms have been prepared using various methods [1] , [2] . The reduced metal atoms are stabilized on solid surfaces through metal-support interaction [3] , [4] or by strong ligand coordination [5] , [6] . The noble metal atoms are often capable of activating adsorbed reactants in catalysis [7] , [8] . Reduced single atoms tend to aggregate into nanoparticles in liquid media in the absence of strong ligand coordination [9] . Full and strong coordination is not desired for metal catalysts [10] . Therefore, synthesis of weakly coordinated and yet stable metal atoms in liquid media may pave a new path for facile preparation of highly dispersed metal catalysts by overcoming the long-standing challenge of metal aggregation. The readily removable ligands from the discrete metal atoms may also potentially enable atomically controllable synthesis of metallic materials by design. Numerous surfactants with diverse functionalities have been used in the synthesis of metallic nanoparticles [11] , [12] or metal ion-surfactant complexes [13] , [14] in micro-emulsions system. The synthesis of discrete reduced metal atoms with weak coordination, which are sufficiently stable in storage at moderate temperature has not been reported. In this work, we chose polydimethylsiloxane-polyethylene glycol (PDMS-PEG) copolymer as an amphiphilic solvating agent. The hydrophilic and semicrystalline PEG blocks enable the dispersion of the hydrophobic PDMS blocks in aqueous solutions [15] , [16] . In our synthesis, ethanol is used as the reductant for Pt(IV) [17] , [18] , in the presence of optimized 10% (v/v) water to accelerate the rate of reduction [9] , while the diverse oxygen-containing functionality of PDMS-PEG offer weak coordination to the Pt atoms. Formation and spectroscopic characterizations of Pt 1 (0) in ethanol reduction of ionic Pt precursors Weakly coordinated mononuclear Pt 1 (0) (Pt 1 @PDMS-PEG) was prepared by ethanol reduction of H 2 PtCl 6 in PDMS-PEG/ethanol−water (see Methods). The characteristic ultraviolet (UV)–visible (Vis) absorption peak of [PtCl 6 ] 2− at 265 nm disappeared and that of [PtCl 4 ] 2− anions at 220 nm was absent [17] , [18] after the solution was refluxed for 3 h at 105 °C, indicating complete reduction of the Pt ions (Fig. 1a ). While the decrease of the signal at 329 cm −1 in far infrared spectra [19] , [20] (Fig. 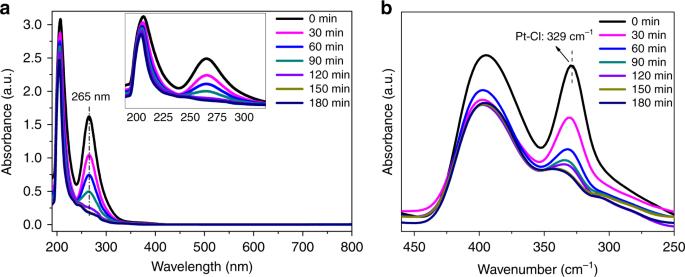Fig. 1 The reduction of H2PtCl6.aUltraviolet (UV)–visible (Vis) spectra of H2PtCl6during the ethanol reduction process.bFar infrared spectra in the process of H2PtCl6reduction 1b ) confirmed the loss of Coulombic Pt–Cl bonds, characterized by the chlorides of positively charged Pt ions, the retained Cl with a Cl/Pt atomic ratio of 2 in Pt 1 @PDMS-PEG was determined by chloride ion-chromatography analysis (Supplementary Table 1 ). 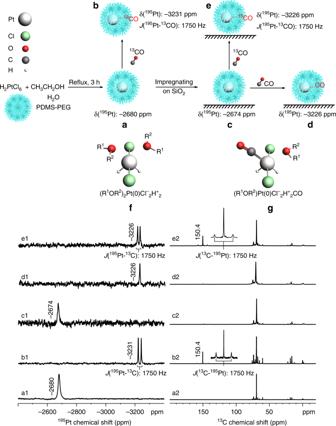Fig. 2 195Pt NMR (a1–e1) and corresponding13C NMR (a2–e2) spectra ofaPt1@PDMS-PEG liquid;b13CO treated Pt1@PDMS-PEG liquid;c2 wt% Pt1@PDMS-PEG/SiO2;dCO treated 2 wt% Pt1@PDMS-PEG/SiO2;e13CO treated 2 wt% Pt1@PDMS-PEG/SiO2. Note: 2 wt% refers to the Pt loading on SiO2;f,gare the selected density functional theory (DFT) models ofpseudooctahedral structure of (R1OR2)2Pt(0)Cl−2H+2(R1, R2are H, C, or Si groups) and (R1OR2)Pt(0)Cl−2H+2CO in polydimethylsiloxane-polyethylene glycol (PDMS-PEG), respectively. Note: the sketch only serves as an illustration of possible local structures Concomitant with the reduction of Pt(IV) (Supplementary Table 2 ), the color of the solution turned from bright yellow to colorless. Furthermore, the characteristic broad peak of Pt nanoparticles between 400 and 800 nm was not observed (Fig. 1a ), indicating the absence of Pt n clusters in the system [21] . When PDMS-PEG was replaced by either PDMS or PEG alone, a dark brown color indicative of Pt nanoparticle formation was observed under the same conditions [18] . Fig. 1 The reduction of H 2 PtCl 6 . a Ultraviolet (UV)–visible (Vis) spectra of H 2 PtCl 6 during the ethanol reduction process. b Far infrared spectra in the process of H 2 PtCl 6 reduction Full size image The absence of 195 Pt nuclear magnetic resonance (NMR) signals near 0 ppm [22] , [23] for [PtCl 6 ] 2− and −1617 ppm [24] for [PtCl 4 ] 2− confirms the full reduction of platinum. Meanwhile, a pronounced 195 Pt NMR peak at −2680 ppm (Fig. 2a 1) was observed and assigned to Pt 1 (0) in PDMS-PEG. This conclusion has been independently verified by the reduction of [PtCl 4 ] 2− in PDMS-PEG monitored by 195 Pt NMR (Supplementary Fig. 1 ). 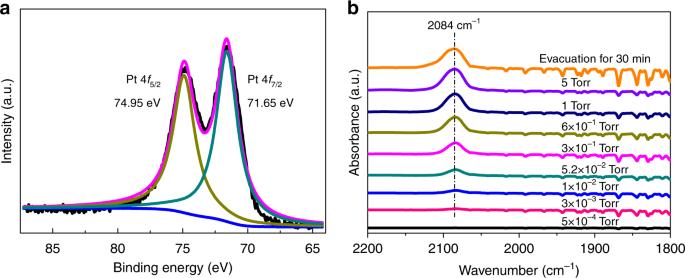Fig. 3 X-ray photoelectron spectra and CO adsorption of Pt1(0) atoms.aX-ray photoelectron spectra of 0.5 wt% Pt1@PDMS-PEG/SiO2, andbIn situ diffuse reflectance infrared Fourier-transform (DRIFT) spectroscopy of CO adsorption on 1 wt% Pt1@PDMS-PEG/SiO2 195 Pt NMR calculation of Pt(II) in PtCl 2 L 2 or binuclear Pt 2 (μ-Cl) 2 Cl 2 L 2 complexes with bridging Cl ligands (Supplementary Table 3 ) also supports the reduced state of Pt 1 center [25] . Fig. 2 195 Pt NMR (a1–e1) and corresponding 13 C NMR (a2–e2) spectra of a Pt 1 @PDMS-PEG liquid; b 13 CO treated Pt 1 @PDMS-PEG liquid; c 2 wt% Pt 1 @PDMS-PEG/SiO 2 ; d CO treated 2 wt% Pt 1 @PDMS-PEG/SiO 2 ; e 13 CO treated 2 wt% Pt 1 @PDMS-PEG/SiO 2 . Note: 2 wt% refers to the Pt loading on SiO 2 ; f , g are the selected density functional theory (DFT) models of pseudo octahedral structure of (R 1 OR 2 ) 2 Pt(0)Cl − 2 H + 2 (R 1 , R 2 are H, C, or Si groups) and (R 1 OR 2 )Pt(0)Cl − 2 H + 2 CO in polydimethylsiloxane-polyethylene glycol (PDMS-PEG), respectively. Note: the sketch only serves as an illustration of possible local structures Full size image CO has been widely used to probe the dispersion of Pt particles on supports [4] . CO is known to coordinate to Pt by forming a linear Pt–CO bond or bridged bonds (Pt 2 CO and Pt 3 CO) on the surface of Pt clusters [4] . The identity of the discrete mononuclear state of Pt atoms was further verified by CO coordination using 195 Pt and 13 C NMR spectroscopy. 13 CO treatment of Pt 1 @PDMS-PEG (Methods) led to an up-field shift of the 195 Pt peak from −2680 to −3231 ppm as a doublet with a splitting of 1750 Hz, (Fig. 2b 1), corresponding to one CO coordination to one Pt 1 (0) center. The 13 C NMR spectrum (Fig. 2b 2) of this sample also showed a new peak at 150.4 ppm with a 195 Pt satellite doublet ( 195 Pt- 13 C O) having the same splitting (1750 Hz). Since the 13 C NMR chemical shift of solvated CO in various solvents ranges from 184.9 to 188.0 ppm [26] , the peak at 150.4 ppm can be assigned to the carbon of the newly formed Pt•••C = O species. In concert with the experimental observation, the density functional theory (DFT) calculation of 13 C NMR chemical shift also shows a 24.1 ppm up-field shift from the gas phase CO to Pt•••C = O (Entries 8, 13 in Supplementary Table 4 ). In both 195 Pt and 13 C NMR spectra, the splitting of 1750 Hz can be unambiguously assigned as the spin–spin coupling constant 1 J ( 195 Pt- 13 C). 13 CO coordination to any form of multi-nuclear platinum cluster would produce more complex spin–spin coupling patterns than a simple doublet (Fig. 2b ) of a linear Pt•••C = O structure. Thus, we conclude that the observed 195 Pt NMR data unambiguously demonstrate the discrete mononuclear state of Pt atoms and Pt 1 •••C = O species, respectively. When a concentrated Pt 1 @PDMS-PEG solution was purged with CO (Methods), a new peak at 341 cm -1 (vibration of Pt 1 -CO) in far infrared appeared [19] , [20] (Supplementary Fig. 2 ). Altogether with the 195 Pt NMR signal shift to −3231 ppm after the 13 CO treatment, the results indicate that CO is a strong ligand. The 195 Pt NMR linewidth of 265 Hz for Pt 1 •••C = O, almost fivefold reduction from that of solvated Pt 1 @PDMS-PEG, may be attributed to the enhanced mobility in the vicinity of Pt sites upon formation of the Pt•••C = O bond. Determination of coordination structure and electronic state of Pt 1 (0) Extensive DFT-based structure screening using geometry optimization was followed by validation through comparing the calculated 195 Pt chemical shifts of the selected structural models [27] , [28] , [29] with the experimental shifts. Consistent with the fact that there are two chlorines per Pt 1 (0) in Pt 1 @PDMS-PEG based on the chloride ion chromatographic analysis, the DFT survey reveals a set of pseudo octahedral structures (R 1 OR 2 ) 2 Pt(0)Cl − 2 H + 2 (R 1 , R 2 are H, C, or Si groups) (Entries 2–5, Supplementary Table 4 ) that not only stabilize Pt 1 (0), but also leads to the calculated 195 Pt chemical shifts in reasonable agreement with the experimental value (−2680 ppm) for Pt 1 @PDMS-PEG. In general, these structures contain two electron-donating oxygens (hydroxyl oxygens of water, ethanol as well as ester oxygens of siloxane and PEG segments) and an otherwise cis -divacant octahedral structure (Pt 1 H 2 Cl 2 ) (Entry 1, Supplementary Table 4 ). The DFT calculation indicates the coordination of Pt 1 (0) by H, Cl, and O simultaneously prevents Pt 1 (0) from forming aggregates. We noted that various oxygen coordinated structures, excluding Cl and H and the structures in which H + bound to Cl − failed to produce a structure matching the observed 195 Pt chemical shift (Supplementary Table 4 ). Moreover, the DFT calculation shows that the Bader charge of Pt atoms in the optimized structures (Entries 1–5, Supplementary Table 4 ) is around 0.6 eV, indicating the Pt 1 (0) atoms are electron deficient (Pt 1 δ+ (0 < δ < 1)), possibly associated with the partial electronegative charge of Cl − . The Bader charge of hydrogen is positive for all optimized (R 1 OR 2 ) 2 PtCl 2 H 2 structures (Entries 2–5, Supplementary Table 4 ), suggesting the H in (R 1 OR 2 ) 2 PtCl 2 H 2 is similar to labile proton rather than to hydride in nature. In the presence of abundant protons such as in residual H 2 O and OH groups of the solvent, the protic H in the (R 1 OR 2 ) 2 PtCl 2 H 2 could be readily hydrated, e.g. H 3 O + . The calculated 195 Pt chemical shift (−2705 ppm) of (R 1 OR 2 ) 2 Pt(0)Cl − 2 (H 3 O + ) 2 (Entry 6, Supplementary Table 4 ) is in an excellent agreement with the experimental shift (−2680 ppm), suggesting that (R 1 OR 2 ) 2 Pt(0)Cl − 2 (H 3 O + ) 2 may exist as a hydrated form of (R 1 OR 2 ) 2 PtCl − 2 H + 2 in the system. This calculated result is a further validation of the existence of protic H, rather than a hydride. The absence of 195 Pt- 1 H spin–spin couplings in the 195 Pt spectra may be explained by the rapid chemical exchanges between the protic H in (R 1 OR 2 ) 2 PtCl - 2 H + 2 and abundant labile protons of water and hydroxyl protons in the system. Furthermore, the protic H in the (R 1 OR 2 ) 2 Pt(0)Cl 2 H 2 is consistent with a recent report that showed HCl acted as a weak ligand in the stabilization of Ir nanoparticles with the H in protic state [30] . The PtCl 2 2− species quickly aggregated to form Pt nanoparticles in methanol−water solution [9] . In our system, the (R 1 OR 2 ) 2 Pt(0)Cl − 2 H + 2 is well stabilized by the PDMS-PEG matrix. Besides the weak coordination of the dioxygen in the liquid, the (R 1 OR 2 ) 2 Pt(0)Cl 2 H 2 is acidic because of the protic H. We found that the Cl and H in PtCl 2 H 2 are readily removable by neutralization with a base, accompanying with the release and subsequent destabilization of bare Pt 1 δ+ atoms even at ambient temperature. The sintering of Pt under such condition was evidenced by noting the color of the solution changing from colorless to dark brown, which apparently is not associated with Pt(II or IV) chlorides. The fact that no redox reaction occurred during the neutralization process confirmed the Pt 1 in (R 1 OR 2 ) 2 PtCl 2 H 2 was in reduced state. The Pt coordination with H and Cl further verified by HBr exchange, which led an up-field 195 Pt NMR chemical shift of (R 1 OR 2 ) 2 PtBr − 2 H + 2 to −3399 ppm (Supplementary Fig. 3 ), as was predicted by the calculated 195 Pt NMR value (−3197 ppm, Entry 7, Supplementary Table 4 ). To further verify the pseudo octahedral structures with a CO coordination as Pt•••C = O, we replaced one of oxygen-containing groups (R 1 OR 2 ) with CO, followed by DFT geometry optimization and 195 Pt NMR chemical shift calculation. The corresponding optimized structures (Entries 9–12, Supplementary Table 4 ) yielded the calculated 195 Pt chemical shifts again in acceptable agreement with the experimental value (−3231 ppm) of Pt•••C = O. A model without proper oxygen coordination (Entry 8, Supplementary Table 4 ) failed to produce 195 Pt chemical shift in conformity to the experimental value. Experimentally, the 195 Pt chemical shift is up-field shifted by 551 ppm from Pt 1 @PDMS-PEG to the CO treated Pt 1 @PDMS-PEG. 195 Pt chemical shift calculation shows that one CO coordination replacing one of the two R 1 OR 2 coordination (Entries 9–12, Supplementary Table 4 ) led to an up-field shift ranging from 366 to 489 ppm compared to the corresponding dioxygen coordinated structures (Entries 2–5, Supplementary Table 4 ), in remarkable agreement with the experimental up-field shift value of 551 ppm. At the same time, replacing the first R 1 OR 2 group with CO is energetically favored (Δ E = −0.18 eV). Further replacement of the remaining R 1 OR 2 with a CO resulted in negligible energy difference (Δ E = −0.04 eV), consistent with fact that only one CO binds to Pt 1 δ+ atom. DFT calculation also shows that di-coordinated Pt(II) structures, trans -Pt(II)Cl 2 (CO) 2 and cis -Pt(II)Cl 2 (CO) 2 , could not produce predicted chemical shifts in agreement with the experimentally observed value −3231 ppm (Supplementary Table 5 ). In addition, unlike (R 1 OR 2 )Pt(0)Cl 2 H 2 , the formation of dicarbonyl complex, Pt(II)Cl 2 (CO) 2 , from Pt(II)Cl 2 (R 1 OR 2 ) is energetically favorable by the DFT calculations (Supplementary Table 5 ). To demonstrate the versatility of preparing supported mononuclear electron-deficient Pt from the liquid Pt 1 (0) precursor, a Pt 1 @PDMS-PEG/SiO 2 sample with Pt loading equivalent to 2.0 wt% with respect to SiO 2 was prepared (see Methods). In comparison, a low Pt loading, e.g., 0.17 wt%, was essential for the direct preparation of Pt single atoms on oxides support [4] to minimize Pt sintering due to its weak interaction with the support. Solid-state 195 Pt magic angle spinning (MAS) NMR spectrum (Figure 2c 1) of the Pt 1 @PDMS-PEG/SiO 2 showed a peak at −2674 ppm, resembling that of Pt 1 @PDMS-PEG in terms of chemical shift. After CO treatment (see Methods), the 195 Pt peak was shifted up-field to −3226 ppm (Figure 2d 1). The same 1 J ( 195 Pt- 13 C) values were simultaneously observed in the 195 Pt and 13 C MAS NMR spectra (Figs. 2e1 and e2 ) upon 13 CO treatment of the Pt 1 @PDMS-PEG/SiO 2 sample, indicating that Pt 1 @PDMS-PEG was well preserved and stably dispersed on the silica surface even after “drying” under vacuum at 40 °C. Remarkably, the Pt 1 @PDMS-PEG and Pt 1 @PDMS-PEG/SiO 2 samples remained stable for over six months in storage at ambient temperature as evidenced by almost identical 195 Pt NMR spectra periodically measured. To further verify the oxidation state of Pt after the reduction, a Pt 1 @PDMS-PEG liquid sample impregnated on pristine SiO 2 was studied by X-ray photoelectron spectroscopy (XPS) (Fig. 3a ). A peak at 71.65 eV (Pt 4 f 7/2 ), which is 0.45 eV higher than that of bulk Pt metal (71.20 eV) [31] and 1.55 eV lower than that of Pt(II) (73.20 eV) [32] , confirmed the reduced state of Pt atoms in Pt 1 @PDMS-PEG/SiO 2 . Only one infrared (IR) absorption peak at 2084 cm −1 was observed for CO adsorbed on Pt 1 @PDMS-PEG/SiO 2 , but not on PDMS-PEG/SiO 2 (Supplementary Fig. 4 ) by in situ diffuse reflectance infrared Fourier-transform (DRIFT) spectroscopy (Fig. 3b ). Peak between 1800 and 1900 cm −1 for bridged CO was not observed, and the peak at 2084 cm −1 did not shift with increasing CO pressure, indicating the absence of nanoparticles in the system [4] . The DRIFT result is consistent with the NMR results of CO treated Pt 1 @PDMS-PEG (one-to-one coordination between CO and Pt 1 δ+ center), and the characteristic peaks at 2178 and 2138 cm -1 corresponding to the cis -Pt(II)Cl 2 (CO) 2 were absent [33] . Fig. 3 X-ray photoelectron spectra and CO adsorption of Pt 1 (0) atoms. a X-ray photoelectron spectra of 0.5 wt% Pt 1 @PDMS-PEG/SiO 2 , and b In situ diffuse reflectance infrared Fourier-transform (DRIFT) spectroscopy of CO adsorption on 1 wt% Pt 1 @PDMS-PEG/SiO 2 Full size image The morphology of Pt 1 @PDMS-PEG solution was characterized by transmission electron microscopy (TEM). Fairly unilamellar vesicles with a narrow distribution (30–80 nm, Supplementary Fig. 5a ) were formed [34] . The energy-dispersive X-ray spectroscopy analysis in a scanning transmission electron microscope (STEM) revealed the existence of Pt in the vesicles (Supplementary Fig. 5b and Supplementary Table 6 ). It should be noted that the Pt atoms tend to agglomerate under intense electron beam or X-ray radiation, making TEM, STEM, and synchrotron X-ray measurements infeasible in providing unambiguous evidence of discrete Pt atoms in our system [35] . Catalytic performance of electron deficient Pt 1 (0) in hydrosilylation reactions An application of Pt 1 @PDMS-PEG as demonstrated in this work is its superb performance in hydrosilylation reaction [36] , [37] . Pt 1 @PDMS-PEG exhibited an ultrahigh activity with high selectivity (99%) to the terminal adduct in the benchmark hydrosilylation reaction of 1-octene and (Me 3 SiO) 2 MeSiH (Supplementary Table 7 and Supplementary Fig. 6 ). No 1-octene conversion was observed in a blank test using PDMS-PEG alone (Supplementary Table 7 ). The turnover frequency (TOF) of the Pt 1 @PDMS-PEG catalyst is 2 to 4 orders of magnitude higher than that of Karstedt [38] , NHC-Pt complexs [37] , [39] , and silylene-Pt complexs [38] , [40] (Supplementary Table 7 and Supplementary Fig. 7 ). The turnover number (TON) exceeded 5.0 × 10 8 for the hydrosilytion reaction of 1-octene using (Me 3 SiO) 2 MeSiH as the silylation reagent. Induction period of the hydrosilylation by Pt 1 @PDMS-PEG was negligible. The reaction solution remained colorless and transparent throughout hydrosilylation reaction. The ultrahigh activity of Pt 1 @PDMS-PEG catalyst may be attributed to electron deficiency of the Pt 1 δ+ center [41] and the reversible weakly electron-donating R 1 OR 2 ligands as compared to the 1,3-divinyl−1,1,3,3-tetramethyldisiloxane (dvtms) or other olefin ligands. The Bader charge (~0.6 eV) on the Pt 1 δ+ center in (R 1 OR 2 ) 2 PtCl 2 H 2 (Entries 2–5, Supplementary Table 4 ) is much higher than the charge (0.13 eV) for Pt in the tri-olefin coordinated complex (Entry 9, Supplementary Table 8 ), representing Karstedt Pt catalyst. 195 Pt chemical shift of the Pt 1 @PDMS-PEG is about 3450 ppm down-field shifted to that of the Karstedt Pt catalyst [42] , also in conformity with the high electron deficiency of the Pt 1 @PDMS-PEG catalyst. The dvtms coordinated Pt catalysts are typically characterized by a relative long induction period partly due to the slow substitution of dvtms by reactants [39] . When 1-octene was added to Pt 1 @PDMS-PEG, the 195 Pt NMR peak showed an insignificant up-field shifted by only 26 ppm to −2706 ppm (Supplementary Fig. 8 ). DFT calculation shows that only mono-olefin complex (olefin) 1 (R 1 OR 2 ) 1 PtCl − 2 H + 2 produces a 195 Pt NMR chemical shift that reasonably agrees with the experimentally observed value (Entry 2, Supplementary Table 8 ). All structures with multiple olefin coordination fail to predict the experimental 195 Pt NMR chemical shift. The dvtms stabilized Pt catalysts were reported to form colloidal platinum species, accompanied by the change of the solution color to yellow during the hydrosilylation catalysis process [43] , [44] , making the nuclearity of the active Pt catalyst debatable. In this work, in addition to the invariant color throughout the hydrosilylation reaction, the 195 Pt NMR of the reaction solution after the catalytic reaction shows that the catalyst remained in mononuclear Pt 1 (0) state (Supplementary Fig. 9 , n 1-octene : n silane = 5:3), suggesting that the highly durable mononuclear Pt 1 (0) center is the active site in Pt 1 @PDMS-PEG for the reaction. Moreover, through three recycled uses, Pt 1 @PDMS-PEG maintained high activity without noticeable deactivation in 1-octene hydrosilylation with (Me 3 SiO) 2 MeSiH (Supplementary Fig. 10 ). The color of the reused Pt 1 @PDMS-PEG solution remained clear throughout the reuses. Conclusion We prepare discrete Pt 1 @PDMS-PEG through ethanol reduction of H 2 PtCl 6 . UV–Vis, Fourier-transform infrared spectroscopy (FTIR), 195 Pt, and 13 C NMR and XPS spectroscopies provide strong evidence for the formation of Pt 1 (0). Based on the extensive DFT structure screening and by comparing the calculated and experimental 195 Pt NMR chemical shifts, a pseudo octahedral Pt 1 (0) structure, (R 1 OR 2 ) 2 Pt(0)Cl − 2 H + 2 with weakly coordinated Pt 1 (0) is proposed. Pt 1 @PDMS-PEG shows high thermal stability in solution and on support in a moderate temperature range. As a catalyst, it exhibits ultrahigh activity and durability for hydrosilylation with superb selectivity to terminal adduct. The electron-deficient Pt 1 δ+ center together with weak oxygen coordination may contribute to the high performance in hydrosilylation. Pt 1 @PDMS-PEG could be a potential new generation of hydrosilylation catalyst. Chemicals 1-Octene (98%), silica, and PEG-200 were purchased from Aladdin Industrial Corporation. PDMS-2000 were purchased from Alfa Aesar (China) Chemicals Co., Ltd. N , N -dimethylaniline (99%) and 1,1,1,3,5,5,5-heptamethyltrisiloxane (98%) were purchased from Tokyo Chemical Industrial Co., LTD. Hydrochloric acid, chloroplatinic acid, ethanol, and ammonium hydroxide were purchased from Sinopharm Chemical Reagent Co., Ltd. PDMS-PEG was purchased from Guangzhou Tinci Materials Technology Co., Ltd. The molecular weight of each block is 30,000 for PDMS and 545 for PEG-12. Ultrapure water purified by Milli-Q Advantage A10 was used. Sample preparation Preparation of Pt 1 @PDMS-PEG stock solution by reduction of H 2 PtCl 6 with ethanol: PDMS-PEG (0.6465 g), ethanol (135 ml), and ultrapure water (10.2 ml) were stirred in a round-bottom flask at 450 rpm at room temperature (RT). After 10 min, 4.8 ml H 2 PtCl 6 solution (1.84 × 10 −2 mol l −1 ) was added, and the mixture was stirred for 10 more minutes. The solution was refluxed at 105 °C for 3 h and then cooled to RT. (For NMR characterization, ethanol and water were evaporated at 40 °C under reduced pressure). 13 CO treatment of Pt 1 @PDMS-PEG: Ethanol and water were removed under vacuum from the Pt 1 @PDMS-PEG stock solution at 40 °C. The Pt 1 @PDMS-PEG sample was purged with He for 30 min (100 ml min −1 ), followed by admission of 5% 13 CO/He (15 ml min −1 ) for another 30 min. The sample was flushed with He for 1 h to remove free 13 CO and collected in a glovebox under N 2 . CO treatment of Pt 1 @PDMS-PEG for Far-IR (FIR) characterization: Ethanol and water were removed under vacuum from the Pt 1 @PDMS-PEG stock solution at 40 °C. The Pt 1 @PDMS-PEG sample was purged with He for 30 min (100 ml min −1 ), followed by admission of 5% CO/He (15 ml min −1 ) for another 30 min. The sample was flushed with He for 1 h to remove free CO and collected in a glovebox under N 2 before the FIR characterization. Preparation of Pt 1 @PDMS-PEG/SiO 2 : A calculated amount of silica based on the desired final Pt loading was added to 150 ml Pt 1 @PDMS-PEG stock solution and stirred for 1 h. Ethanol and water were removed at 40 °C under vacuum. The sample was further vacuum dried for 12 h at 40 °C. For DRIFT experiment and catalytic reactions, the pH value of the Pt 1 @PDMS-PEG stock solution was adjusted to 3.2 by NH 3 •H 2 O solution before the evacuation. 13 CO treatment of Pt 1 @PDMS-PEG/SiO 2 : In a quartz tube 200 mg Pt 1 @PDMS-PEG/SiO 2 was purged with He for 30 min (100 ml min −1 ) and 5% 13 CO/He (15 ml min −1 ) for another 30 min. The sample was flushed with He for 1 h to remove free gas phase 13 CO and collected in a glovebox under N 2 . 1-Octene disposed Pt 1 @PDMS-PEG: Concentrated 150 ml Pt 1 @PDMS-PEG solution to 20 ml. Added 0.0990 g 1-octene (ten times equivalent to Pt 1 ) and 6 ml CHCl 3 into the 20 ml concentrated solution (the use of CHCl 3 is to enhance the 1-octene dissolution in the system). Stirred for 24 h at 40 °C and followed by further concentrating the solution to about 3 ml. The sample was collected in a glovebox under N 2 prior to the 195 Pt NMR measurement. Ultraviolet (UV)–visible (Vis) UV–Vis spectra was collected on a Shimadzu UV-2600 spectrophotometer. X-ray photoelectron spectra (XPS) The surface composition and the binding energy (B.E.) of the catalyst were determined by XPS on an ESCALAB250 X-ray photoelectron spectrometer with contaminated C as the internal standard (C1s = 284.6 eV). NMR spectroscopy All solid-state NMR measurements were carried out on a 11.7 T wide-bore Bruker Avance III solid-state NMR spectrometer, operating at a Larmor frequency of 500.13 MHz for 1 H, 125.77 MHz for 13 C, and 107.21 MHz for 195 Pt. A 4.0 mm Bruker multinuclear HX double resonance magic angle spinning (MAS) probe was used. The experiments were acquired at 25 °C and an MAS frequency of 10 kHz, controlled to within +/−3 Hz using the Bruker MAS controller. The typical 90° pulse length was 2.5 μs ( 1 H), 3.6 μs ( 13 C), and 4.2 μs ( 195 Pt). Seventy-six thousand two-hundred scans were collected for 195 Pt MAS NMR spectra with a recycle delay of 1 s and 30° pulse excitation (1.4 us). Eight-thousand one-hundred ninety-two scans were collected for 13 C MAS NMR spectra with a recycle delay of 3 s, where 1 H SPINAL-64 heteronuclear decoupling with field strength of 90 kHz was applied during the acquisition period. Solution NMR spectra were obtained on Bruker Avance III 600 MHz and 400 MHz using the 5 mm multinuclear probe. Single pulse and proton decoupling were used for 195 Pt and 13 C measurements with 3-s relaxation delay, respectively. The solution and solid-state 195 Pt NMR spectra were referenced to a platinum peak of a 1.2 M Na 2 PtCl 6 D 2 O solution. The chemical shifts of 1 H and 29 Si NMR spectra were referenced externally to TMS. Fourier-transform infrared spectroscopy (FTIR) A DiffusIR diffuse reflectance accessory (Pike Technologies) was used for the FTIR measurements. A leveled attenuated total reflectance (ATR) accessory (Pike Technologies) with a 3 mm diameter diamond plate was used for Middle IR (MIR) and FIR measurements. The FIR instrument (Thermo Scientific Nicolet iS50) is equipped with mercury cadmium telluride (MCT) detector and DTGS/polyethylene detector. The DRIFT measurement has a resolution of 4 cm −1 and 64 scans were collected, while for FIR measurements, 128 scans were collected with a resolution of 16 cm −1 . For the DRIFT measurements, the sample was evacuated at 25 °C for 1 h before absorption of high purity probing CO gas. For the FIR measurements, a steady flow of nitrogen was maintained and a high-temperature vacuum-grease-sealed glass lid was used above the sample to prevent air and moisture. Before the FIR experiment, ethanol and water in all the samples were removed by evacuation. Transmission electron microscopy (TEM) and scanning transmission electron microscope (STEM) STEM analyses were performed with a JEOL JEM-2100F microscope operated at 200 kV. TEM analyses were performed with a JEOL JEM-2000EX microscope operated at 120 kV. A few droplets of the stock solution were put on a microgrid carbon polymer supported on a copper grid and allowed to dry out at room temperature for TEM and STEM observations. The samples were evacuated under ultrahigh vacuum for 20 min in the microscope before observations. For TEM characterization, phosphotungstic acid was used as the staining reagent. Chloride ion analysis by ion-chromatography A THERMOICS-5000 ion-chromatography with the Electrochemical Detector (ED) and the AS-11 and AS-22 columns ware used for the detection of Cl − in Pt 1 @PDMS-PEG. Before detection, a 5 ml of Pt 1 @PDMS-PEG was diluted to 10 ml with water to reach an appropriate concentration for ion chromatographic analysis. Computation of NMR shifts The Amsterdam Density Functional (ADF) approach [45] , by which the relativistic effects for calculating of chemical shielding of heavy atom such as platinum can be implemented, was used. The relativistic effects were treated in the ADF as all-electron zeroth-order regular approximation (ZORA). For the chemical shielding, the spin-orbital (SO) two-component was used while for the geometry optimization the scalar approximation neglecting SO coupling was utilized. More specifically, as suggested by Autschbach et al. [27] , [28] , [29] , the revised Perdew-Burke-Ernzerhof (revPEB) functional was used for all calculations, and the Slate-type of basis sets (TP2Z) were used for ligand atoms and the quadruple-quadruply polarized (QZ4P) ZORA basis was set for Pt, respectively. The calculated chemical shift of the optimized structures was referenced to the calculated isotropic shielding constant ( σ ref = 2005 ppm) of the reference compound [PtCl 6 ] 2− by the definition of δ = ( σ ref − σ )/(1 − σ ref ) ≈ ( σ ref − σ ) with an assumption that (1 − σ ref ) ≈ 1. The geometry of [PtCl 6 ] 2 was optimized ( d Pt-Cl = 2.392 Å) using the same method described above prior to the calculation of the shielding constant ( σ ref ). Similar ADF method with scalar approximation neglecting SO coupling was used to calcuate 13 C chemcial shielding of gas phase CO and Pt-coordinated CO in various structures. General procedure for hydrosilylation We followed Iwamoto’s procedure [38] to evaluate the Pt 1 @PDMS-PEG as the catalyst for the hydrosilylation reaction of 1-octene with 1,1,1,3,5,5,5-heptamethyltrisiloxane (Supplementary Table 7 ). In all, 0.034 ml Pt 1 @PDMS-PEG stock solution (Pt concentration of 5.88 × 10 −4 mol l −1 ) was added into the reactor. Ethanol and water were evacuated at RT. All reactions were carried out in glovebox. 1-Octene (4 mmol) was added and mixed with the Pt 1 @PDMS-PEG [corresponding to n (1-octene): n (Pt 1 ) = 200,000:1] for 3 min at 25 °C before reaction. 1,1,1,3,5,5,5-heptamethyltrisiloxane (4.4 mmol) was then added, and the reaction was carried out at 50 °C. After reaction, 2 mmol N , N -dimethylaniline (0.2424 g) was added as an internal standard. Products and reactants were characterized by 1 H NMR (400 MHz, CDCl 3 , and Supplementary Fig. 6 ). Blank test was run as follows: hydrosilylation reaction was carried out with PDMS-PEG/ethanol-water as the catalyst (without Pt) following the same procedure as for the hydrosilylation of 1-octene catalyzed by Pt 1 @PDMS-PEG, No conversion of 1-octene was observed (Supplementary Table 7 ). The reported conversion measurement was repeated at least three times under the same condition, and the uncertainty was typically below 5%. The average value of multiple measurements is presented in the paper. The turnover frequency (TOF), defined as the number of moles of terminal product ( T ) yield per mole of Pt 1 (0) within a unit time, is calculated in unit of h −1 according to 
    [                         TOF                           =                n_T/n_Pt×1/t;                                                       = n_olefin,0×yield_T/n_Pt×1/t ]
 Since the conversion reached nearly completion in a minute, the initial TOF was calculated by taking t as 1 min for the catalytic reaction under consideration. n olefin,0 is the initial number of moles of 1-octene used in the reaction. Note that n 1−octene,0 is 4 mmol. n T is the number of moles of product, T (terminal adduct). n Pt is the number of moles of Pt added in the reaction. t is the reaction time. The conversion value was calculated at t = 1 min. yield_T = conversion×selectivity
 Turnover numbers (TONs) TON of Pt 1 @PDMS-PEG in the hydrosilylation reaction between 1-octene and 1,1,1,3,5,5,5-heptamethyltrisiloxane: 0.0068 ml Pt 1 @PDMS-PEG stock solution (diluted 10 times, 5.88 × 10 −5 mol l −1 , 4 × 10 −10 mol) was added into the round-bottom flask, followed by evacuation of ethanol-water. All reaction was carried out in glovebox. 1-Octene (40 mmol) was added and mixed with the Pt 1 @PDMS-PEG [ n (1-octene): n (Pt 1 ) = 1 × 10 8 : 1] for 3 min at 25 °C before reaction. 1,1,1,3,5,5,5-heptamethyltrisiloxane (48 mmol) was then added, and the mixture was refluxed at 70 °C. After the completion of the reaction (verified by 1 H NMR), add more 1-octene and 1,1,1,3,5,5,5-heptamethyltrisiloxane (1:1.2) into the reactor and continue the reaction. Catalyst recycle After the hydrosilylation reaction between 1-octene and (Me 3 SiO) 2 MeSiH (1-octene: 0.4488 g, (Me 3 SiO) 2 MeSiH: 0.89 g) finished, the solution was centrifuged. In all, 0.6694 g reaction mixture was taken out from the upper solution, and analyzed by 1 H NMR. The remaining solution (0.6694 g) was used for the subsequent hydrosilylation reaction. For the reuse test, 0.4488 g 1-octene and 0.89 g (Me 3 SiO) 2 MeSiH was added. After reaction, solution was centrifuged. In all, 1.3388 g (equal to the amount of added reactants) reaction mixture was taken out from the upper solution, and analyzed by 1 H NMR, while the remaining solution (0.6694 g) was used for the subsequent hydrosilylation reaction. For the following reuses, the added amounts of 1-octene and (Me 3 SiO) 2 MeSiH were always 0.4488 and 0.89 g, respectively. After each reaction, the amount of reaction mixture taken out for 1 H NMR from the upper solution after centrifugation was always 1.3388 g (equal to the amount of added reactants), and the remaining solution was kept at 0.6694 g for the subsequent hydrosilylation reaction.